A systems approach towards the stoichiometry-controlled hetero-assembly of nanoparticles A central theme in nanotechnology is to advance the fundamental understanding of nanoscale component assembly, thereby allowing rational structural design that may lead to materials with novel properties and functions. Nanoparticles (NPs) are often regarded as 'artificial atoms', but their 'reactions' are not readily controllable. Here, we demonstrate a complete nanoreaction system whereby colloidal NPs are rationally assembled and purified. Two types of functionalized gold NPs (A and B) are bonded to give specific products AB, AB 2 , AB 3 and AB 4 . The stoichiometry control is realized by fine-tuning the charge repulsion among the B-NPs. The products are protected by a polymer, which allows their isolation in high purity. The integration of hetero-assembly, stoichiometry control, protection scheme and separation method may provide a scalable way to fabricate sophisticated nanostructures. Colloidal growth of nanoparticles (NPs) has been a major focus in nanoscience over the past decades. It provides a scalable and versatile approach to control the size and morphology of NPs, which are critical for their properties. NPs with simple geometries, such as spheres, rods, cubes and triangular prisms, have been prepared with excellent control [1] , [2] , [3] , [4] , [5] . In contrast, colloidal assembly of NPs has been less studied, although it could conceivably offer novel synthetic controls for multi-component nanoclusters. The key challenge is to develop general methodologies to assemble colloidal nano-objects with precise stoichiometry. Previously, homo-aggregates such as dimers and trimers were prepared by exploiting either random aggregation [6] , [7] , [8] , steric effects [9] , [10] , [11] , [12] or specific control over surface ligands (for example, divalent NPs) [13] , [14] , [15] , [16] . Compared with these 'homo-coupling' nanoreactions, controlling stoichiometry in the 'cross-coupling' of NPs presents different and arguably greater challenges. It was only achieved through the brilliant design and pre-fabrication of NPs with anisotropic surface functionalities (for example, NP with a single DNA molecule) [17] , [18] , [19] , [20] , [21] , [22] . In a sense, the assembly of NPs in a colloidal solution is analogous to molecular reactions. Rationally controlled organic syntheses, completed with coupling, protection and separation schemes, have given rise to complex molecules with precise structural control. From this perspective, a complete nanoreaction system emulating the concepts and strategies of molecular reactions may offer a systematic approach to sophisticated nanostructures. A major problem in assembling NPs is the preservation of the product nanoclusters against both disintegration and aggregation, which is often exacerbated by ligand dissociation and exchange over long periods of time. We have recently demonstrated that encapsulation of nanoclusters in polystyrene- block -poly(acrylic acid) (PSPAA) micelles is a way to overcome these problems and affords sufficient stability for the nanoclusters to be separated using concentrated CsCl solutions [6] , [23] , [24] . Here, we combine the protection and purification schemes with the hetero-assembly of NPs, making it possible to recover pure nanoclusters with long-term stability. The stoichiometry of the assemblies was controlled by modulating the charge repulsion among the NPs. The systems approach led to nanoreactions with new structural control. We show that this complete nanoreaction system is an ideal platform for studying the interactions of NPs, just as the studies of molecular reactions provide insight to the chemical nature of atoms. Assembly of AB n nanoclusters Two types of NPs were prepared as the basic reactants: group A was gold NPs (AuNPs) coated with a tetrathiol molecule, 1 ( Fig. 1a , giving A-NPs), whereas group B was citrate-stabilized AuNPs (B-NPs; Fig. 2a ). To mimic molecular reactions, it is critical that these two types of NPs could react with each other, but do not form aggregates of their own. The thiol groups of 1 allowed the ligand to firmly anchor on AuNP while presenting extra thiol groups that could bond to additional AuNPs (that is, forming AuNP- 1 -AuNP bridges through the Au-S interactions). Hence, the A-NPs have to be completely covered with 1 , so that they would not provide exposed Au surface for bonding among themselves. These NPs were, thus, synthesized by treating citrate-AuNPs with excess 1 , and the free ligands were then removed by centrifugation. The purified A-NPs were relatively stable in dimethylformamide (DMF), but they were used shortly after the synthesis. In the absence of excess 1 , the A-NPs could undergo partial ligand dissociation, which will lead to aggregation. Finally, the stoichiometry of the NP assemblies has to be controlled. Without restrictions, multiple B-NPs could bond to each A-NP and vise versa , leading to extensive and uncontrolled aggregation of the two reactants ( Supplementary Figs S1 and S2 ). Our strategy here is to treat A-NPs with excess B-NPs, and to control the stoichiometry of the product AB n by fine-tuning the repulsion between the B-NPs. 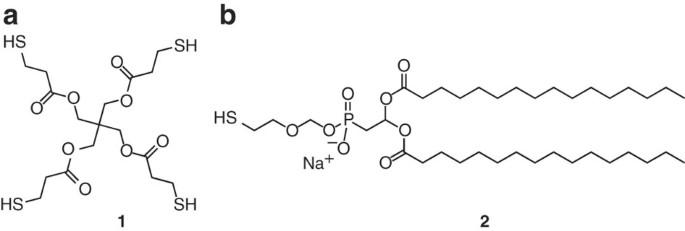Figure 1: Structure of the two ligands used in this study. (a) A tetrathiol ligand, pentaerythritol tetrakis(3-mercapto-propionate) (1). (b) A thiol-ended hydrophobic ligand, 2-dipalmitoyl-sn-glycero-3-phosphothioethanol (sodium salt) (2). Figure 1: Structure of the two ligands used in this study. ( a ) A tetrathiol ligand, pentaerythritol tetrakis(3-mercapto-propionate) ( 1 ). ( b ) A thiol-ended hydrophobic ligand, 2-dipalmitoyl- sn -glycero-3-phosphothioethanol (sodium salt) ( 2 ). 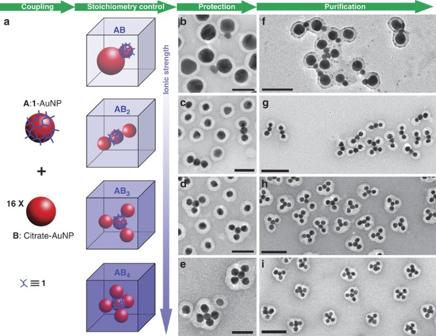Figure 2: Stoichiometry-controlled nanoreactions. (a) Schematics showing the syntheses of AB, AB2, AB3and AB4nanoclusters, by tuning the charge repulsion between the B-NPs (through the ionic strength of the reaction media). The intensity of the shade in the boxes is correlated to the ionic strength of the media: from top down, 0.297, 0.594, 5.04 and 7.29 mM. (b–e) TEM images of the ABnnanoclusters after protection by PSPAA, whereby the nanoclusters were treated with PSPAA and the hydrophobic ligand2. The surface of B-NP is rendered hydrophobic by ligand exchange, on which the PSPAA self-assembles to form a uniform shell. The excess B-NPs are also encapsulated, but the A-NPs are not encapsulated because of persistence of the polar ligand1. SeeTable 1for product analyses. (f–i) TEM images of the purified nanoclusters. Scale bars are 50 nm forb–eand 100 nm forf–i. Full size image Figure 2: Stoichiometry-controlled nanoreactions. ( a ) Schematics showing the syntheses of AB, AB 2 , AB 3 and AB 4 nanoclusters, by tuning the charge repulsion between the B-NPs (through the ionic strength of the reaction media). The intensity of the shade in the boxes is correlated to the ionic strength of the media: from top down, 0.297, 0.594, 5.04 and 7.29 mM. ( b – e ) TEM images of the AB n nanoclusters after protection by PSPAA, whereby the nanoclusters were treated with PSPAA and the hydrophobic ligand 2 . The surface of B-NP is rendered hydrophobic by ligand exchange, on which the PSPAA self-assembles to form a uniform shell. The excess B-NPs are also encapsulated, but the A-NPs are not encapsulated because of persistence of the polar ligand 1 . See Table 1 for product analyses. ( f – i ) TEM images of the purified nanoclusters. Scale bars are 50 nm for b – e and 100 nm for f – i . Full size image In a colloidal reaction, the purified A-NPs in DMF (100 μl, d A =18 nm) was slowly added to an aqueous solution containing large excess of B-NPs (200 μl, d B =18 nm, and final [A]:[B]=1:16; see details in Supplementary Methods ). The random collision between A- and B-NPs gives AB n nanoclusters. However, the product solution cannot be directly characterized by transmission electron microscopy (TEM), as any drying or purification process would lead to significant aggregation of the solution species. Hence, both the product AB n and the remaining B-NPs were protected by PSPAA encapsulation ( Fig. 2b–e ), which basically involved the functionalization of the B-NP surface by a hydrophobic ligand ( 2 , Fig. 1b ), followed by PSPAA self-assembly [6] , [25] , [26] . Ligand 2 cannot replace the hydrophilic ligand 1 on the surface of A-NPs, which was thus not encapsulated. The resulting AB n @PSPAA and B@PSPAA were readily isolated from the preparative solution by centrifugation, and then they were re-dispersed in water. With the polymer protection, the nanoclusters are stable against dissociation and aggregation. This allowed detailed product analysis of the nanoreactions by TEM characterization, giving a window for mechanistic insights. Figure 2c shows the TEM image of a sample that contained trimeric nanoclusters, where the polymer shells only attached to the AuNPs on the ends but not to the central one. The uniformity of this unique polymer coverage ( Fig. 2g ) indicated that the trimeric clusters were not B 3 @PSPAA, but rather (BAB)@PSPAA. This assignment is consistent with the expectations that 2 could replace citrate ions on B-NPs but not the multidentate 1 on A-NPs, and that PSPAA could only attach to regions covered with non-polar and hydrophobic ligands such as 2 (ref. 12 ). Thus, the nanoreaction was successful in giving the AB 2 nanoclusters. The reaction product was surveyed based on the TEM images ( Supplementary Fig. S3 ). As excess B-NPs were used, the yield of the product AB 2 (89.4%, Table 1 ) was calculated based on the number of A-NPs. The by-products included a few AB, AB 3 and also A x B y nanoclusters that may result from aggregated A-NPs. It was intriguing that the nanoreaction terminated at AB 2 despite the presence of excess B-NPs. As a NP in close packing has a coordination number of 12, there was sufficient space on the AB 2 for additional bonding with B-NPs. Obviously, some form of repulsion other than steric hindrance was responsible for the stoichiometry control. As strong electric or magnetic dipoles are unlikely for the large spherical AuNPs (>5 nm) (ref. 27 ), the most likely candidate is charge repulsion. Moreover, the linear AB 2 is reminiscent of the linear aggregates of AuNPs reported earlier [28] , [29] , where charge and dipole interactions were proposed to be the main factors in the geometric control. Table 1 Product analyses of the nanoreactions. Full size table To test this proposal, the colloidal reactions were carried out in solutions with varying ionic strengths ( Table 1 , Supplementary Figs S4 , S5 , S6 , S7 and S8 ), which are known to modulate the charge repulsion between NPs. Although it was difficult to adjust the ionic strength using a single salt owing to the stability requirements for the reactant NPs, it was clear that the size of AB n nanoclusters increased with increasing [Na 3 citrate] or [NaCl] ( Table 1 and Fig. 2 ). In particular, the sole increase of [NaCl] from 0 to 2.25 mM (entry 5 and 6) changed the major product of the nanoreaction from AB 3 (65.6%) to AB 4 (64.9%). In entry 4 of Table 1 , NaNO 3 was shown to have a similar effect as NaCl, indicating that the Cl − ions were not particularly important. Thus, the stoichiometry control of AB n was probably more relevant to the general ionic strength of the solution than other effects. Clear distance existed between the neighbouring B-NPs in all AB n nanoclusters, leading to linear (AB 2 ), triangular (AB 3 ) or tetrahedron (AB 4 ) geometries. Although the large nanoclusters such as AB 3 and AB 4 were often completely engulfed by the polymer shell ( Fig. 2h,i ), their structural uniformity indicated that the hetero-assembly were successful and that the central NPs were all A-NPs. Notably, the ∼ 18 nm separation of the B-NPs in AB 2 is a testament for the strong long-range repulsion during the formation of the nanoclusters. Such a force is most probably charge repulsion. It is hence likely that the increase in ionic strength led to more effective shielding of the surface charges, allowing more B-NPs to bond to each A-NP. Mechanistic analysis of the nanoreactions Interestingly, at low-salt conditions ( Table 1 , entry 1) some heterodimers AB@PSPAA (18.2%) were observed in addition to AB 2 @PSPAA (74.0%; d A = d B =18 nm). The partial polymer coverage demonstrated that these dimers were not B 2 @PSPAA. The fact that the AB nanoclusters only occurred in the low-salt reactions indicated that they probably did not originate from the dissociation of AB 2 . Instead, they could be considered as an intermediate before the formation of AB 2 . Should charge repulsion between the B-NPs be a dominant factor in controlling this nanoreaction, larger B-NPs are expected to trap more AB nanoclusters, owing to their larger size and stronger charge repulsion. As expected, reacting 18 nm A-NPs with 36 nm B-NPs under otherwise similar experimental conditions gave heterodimers AB@PSPAA in excellent yield (90.4%, Figs 2b and 3c ). Synthesis of heterodimers is a major challenge in colloidal assembly. Our simple approach has achieved the same level of specificity as those of DNA-based assembly techniques [20] , [30] . The AB heterodimers could also be categorized as 'Janus' NPs [12] , [31] in that they possess two diametric faces of different chemical functionalities. 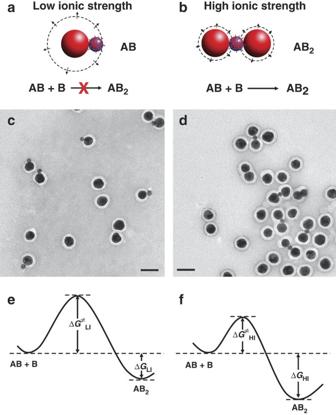Figure 3: Understanding the stoichiometry control in the nanoreactions. (a,b) Schematics showing the syntheses of AB and AB2nanoclusters (dA=18 nm,dB=36 nm). Dashed circles with arrows indicate the strength of charge repulsion; larger radius means stronger repulsion. (c,d) TEM images of the AB and AB2samples after PSPAA protection. All scale bars are 50 nm. (e,f) Schematics showing the reaction coordinates of equation (1) at low and high ionic strengths, respectively. Figure 3: Understanding the stoichiometry control in the nanoreactions. ( a , b ) Schematics showing the syntheses of AB and AB 2 nanoclusters ( d A =18 nm, d B =36 nm). Dashed circles with arrows indicate the strength of charge repulsion; larger radius means stronger repulsion. ( c , d ) TEM images of the AB and AB 2 samples after PSPAA protection. All scale bars are 50 nm. ( e , f ) Schematics showing the reaction coordinates of equation (1) at low and high ionic strengths, respectively. Full size image By increasing ionic strength in this reaction ([NaCl]=3.00 mM), AB 2 @PSPAA (85.7%, Fig. 3d ) resulted instead. These two reactions ruled out electric or magnetic dipoles as the key controlling factors: although it is possible to argue that transient or static dipoles dictate the linear encounter of AB with a B-NP in forming the AB 2 nanocluster ( Figs 2c and 3d ), the dipoles cannot explain the non-reactivity of AB at low ionic strength ( Fig. 3c , and entry 7 of Table 1 ). Any charge–dipole or dipole–dipole interaction would have facilitated the reaction of equation (1) rather than impeding it. Alternatively, long-range (>18 nm) charge repulsion between the B-NPs could best explain the non-reactivity of AB; it is also consistent with the formation of AB 2 at increased ionic strength. Although it is hard to determine the charge of A-NPs, it is clear that the charge interaction between A- and B-NP has a minor role as AB clusters readily formed even at lowest ionic strength. To understand how charge interactions affect the nanoreactions, it is critical to determine whether the reactions are thermodynamically or kinetically controlled. In equation (1), the covalent bonding between A- and B-NPs should be the main driving force for the reaction, although other factors, such as charge–charge interactions ( V elec ), Van der Waals interactions, solvophobic effects and possibly also charge–dipole or dipole–dipole interactions, may contribute to the Δ G . On the other hand, the transition state should occur at a point before the chemical bond formation ( Fig. 3e–f ), where the long-range charge interaction would dominate. Thus, the V elec has to be overcome before effective collision could take place, making it a major contributor of Δ G ≠ . Hence, both Δ G and Δ G ≠ should decrease at high ionic strength owing to weak charge repulsion. This leads to two scenarios that could explain the non-reactivity of AB at low ionic strength. If the reactions are thermodynamically controlled, the kinetic energy (KE) of the NPs should exceed the activation barrier (Δ G ≠ ), whereas ΔG HI (HI stands for high ionic strength) should be <0 at high ionic strength (forward reaction), and ΔG LI >0 at low ionic strength (backward reaction). That is, the system was at or close to equilibrium at the end of reaction and the AB nanoclusters formed because they were the most stable state. In contrast, kinetically controlled reactions would mean that KE>Δ G ≠ HI (forward reaction), but KE <Δ G ≠ LI (no reaction); both ΔG LI and ΔG HI should be <0 in this case. Hence, the AB nanoclusters accumulated, because the KE of the reactants was insufficient to cross the activation barrier to make AB 2 . Experiments were carried out to distinguish these two possibilities. After the formation of AB 3 clusters ( d A = d B =18 nm), the colloid was diluted and incubated in an aqueous solution at low ionic strength (0.297 mM) before PSPAA encapsulation. However, few AB 2 or AB clusters were obtained even when the incubation was carried out at elevated temperature or under sonication ( Supplementary Fig. S9 ). Therefore, it is unlikely that the nanoreactions were reversible. Furthermore, the AB 3 @PSPAA in Figure 2h often deviated from perfect triangles and sometimes appeared in T shape, suggesting the addition of a B-NP to a linear BAB intermediate during its formation. This observation is generally consistent with a non-reversible and kinetically controlled reaction. The electrostatic repulsion potential ( V elec ) between the B-NPs can be estimated by linear superposition approximation [32] , [33] , [34] : where L e = κ −1 is the Debye screening length, calculated from the dielectric constant ϵ of the medium, the Boltzmann constant k , the temperature T , the elementary charge e and the ionic strength I of the electrolyte (equation (3)); a i is the particle radius; h m is the separation distance of the interacting B-NPs; and Ψ i is the surface potential of the particle. Therefore, an increase in the radius of B-NPs results in an increase in a i 2 /(h m +2a i ), and thus, a correspondingly larger repulsion potential V elec . Furthermore, as V elec is proportional to , high ionic strength leads to weak repulsion potential, consistent with the experimental results ( Table 1 ). In Figure 2 , the initial bonding of A-NP and B-NP is favourable, but further attachment of a B-NP on the resulting AB cluster has to overcome the repulsion between the B-NPs, which becomes stronger as the AB n cluster increases in size. At a specific ionic strength, the growth of AB n stops when the KE of the colliding NPs could not exceed the repulsion potential V elec . High ionic strength lowers the V elec , thus allowing more B-NPs to react with each A-NP ( Fig. 2a ). Understandably, the size variation among the A-NPs and B-NPs will cause unequal charge repulsions and thus lead to non-uniformity in the stoichiometry of the product nanoclusters. This is in drastic contrast to molecular reactions where all atoms or molecules are perfectly uniform. Purification To mimic molecular reactions, the products of the nanoreactions have to be purified by removing the excess B@PSPAA. As the overall densities of AB n @PSPAA ( n =2–4) are significantly larger than that of B@PSPAA, the former was easily isolated by differential centrifugation [24] . 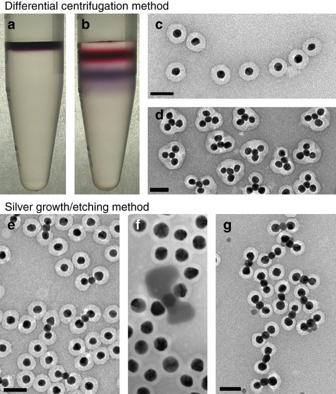Figure 4: Purification of the ABn@PSPAA nanoclusters. (a,b) Photographs of a sample solution before and after differential centrifugation. (c,d) TEM images of the separated B@PSPAA and AB3@PSPAA partitions. (e,f) TEM images of the AB2@PSPAA and B@PSPAA mixture before and after Ag growth on the A-NPs. (g) TEM image of the sample infafter centrifugation and etching Ag. All scale bars are 50 nm. Figure 4a–d shows a typical purification, in which the product solution containing AB 3 @PSPAA was carefully layered on top of a saturated CsCl solution (no concentration gradient was used). After centrifugation, the B@PSPAA and AB 3 @PSPAA were separated into two distinct bands of red and blue colour, respectively. The blue band was enriched in AB 3 @PSPAA, and its colour indicated surface plasmon coupling among the AuNPs of AB 3 . This band was isolated, diluted by aq. NaOH (pH=10) and then centrifuged again to remove the excess CsCl. The purity of the resulting AB 2 -, AB 3 - and AB 4 @PSPAA, as based on the surveys of over 1,000 nanoclusters in TEM images, were 87.3, 64.1 and 67.5%, respectively ( Fig. 2g–i , Supplementary Figs S10 , S11 and S12 ). Most of the impurities in these samples were AB n @PSPAA nanoclusters. The non-ideal purities achieved here could be attributed to the imperfect uniformity in the size of the original AuNPs, which affects both the yield of the nanoreactions and also the efficacy of the purification. Figure 4: Purification of the AB n @PSPAA nanoclusters. ( a , b ) Photographs of a sample solution before and after differential centrifugation. ( c , d ) TEM images of the separated B@PSPAA and AB 3 @PSPAA partitions. ( e , f ) TEM images of the AB 2 @PSPAA and B@PSPAA mixture before and after Ag growth on the A-NPs. ( g ) TEM image of the sample in f after centrifugation and etching Ag. All scale bars are 50 nm. Full size image An alternative method was adapted for the separation of AB- and AB 2 @PSPAA ( Table 1 , entry 2 and 7), in which the exposed A-NPs were exploited as seeds for growing metallic Ag ( Fig. 4e–f , Supplementary Fig. S13 ). In contrast, no Ag growth occurred on the PSPAA shells. As a result, the AB 2 @PSPAA grew significantly heavier than the fully encapsulated B@PSPAA, and they could be easily isolated from the latter by centrifugation at low speed in water. Subsequently, the isolated Ag-(AB 2 @PSPAA) were washed with NH 3 ·H 2 O to etch the Ag blocks, and then centrifuged to remove the excess reactants ( Fig. 4g ). Using this method, AB 2 @PSPAA were isolated in 85.9% purity ( Supplementary Fig. S14 ). This technique was essential for the purification of AB@PSPAA ( Fig. 2f , purity 83.2%, d A =18 nm, d B =36 nm), as there was only a small density difference between the AB- and B@PSPAA ( Supplementary Figs. S15 and S16 ). As such, it is nearly impossible to separate them by the differential centrifugation method. For AB 3 - and AB 4 @PSPAA, however, the polymer shell tends to enclose the whole nanoclusters without exposing the A-NPs; this prevents Ag attachment and thus renders the purification method ineffective. Hence, the two purification methods are complementary in recovering the nanoreaction products and may allow flexibility in designing future synthetic routes. So far, in our nanoreactions, the size of the B-NPs is always larger than or equal to the size of A-NPs. This setup effectively used the charge repulsion between B-NPs for the stoichiometry control. Reacting large A-NPs (36 nm) with small B-NPs (18 nm) is also feasible ( Fig. 5 , Supplementary Figs S17 and S18 ). However, the stoichiometry of the resulting nanoclusters was less uniform, most likely because of the fact that the repulsion between B-NPs was not far enough to affect all neighbours on the large surface of A-NPs. Nevertheless, controlling the ionic strength still by and large controlled the stoichiometry of the AB n nanoclusters. 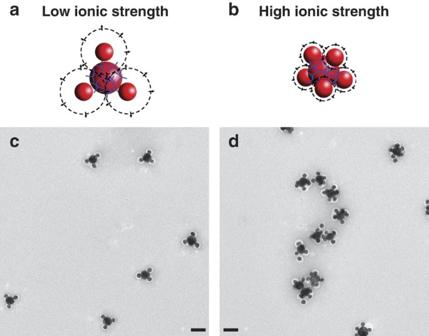Figure 5: TEM images of the ABnnanoclusters (dA=36 nm,dB=18 nm). (a) Nanoreaction carried out at a low ionic strength (I=0.594 mM); (b) nanoreaction carried out at a high ionic strength (I=3.30 mM). (c,d) TEM images of the resulting nanoclusters of (a) and (b), respectively. All scale bars are 50 nm. Figure 5: TEM images of the AB n nanoclusters ( d A =36 nm, d B =18 nm). ( a ) Nanoreaction carried out at a low ionic strength ( I =0.594 mM); ( b ) nanoreaction carried out at a high ionic strength ( I =3.30 mM). ( c , d ) TEM images of the resulting nanoclusters of ( a ) and ( b ), respectively. All scale bars are 50 nm. Full size image We demonstrated a systems approach to colloidal assembly of Au NPs. By understanding and directing the reaction kinetics, the stoichiometry of the product nanoclusters was controlled simply by modulating the ionic strength of the reaction media. Colloidal synthesis is generally scalable and easy to control; and the polymer protection led to the recovery of pure nanoclusters with long-term stability. Hence, this initial platform of NP-based reactions permits further development of synthetic methodologies. In addition, the well-controlled reactions also allow insights into the interactions of NPs. Specifically, charge repulsion has been identified as the major factor in the stoichiometry control in our system, whereas charge or magnetic dipoles were ruled out. The nanoreactions were found to be kinetically controlled: the reaction proceeds at high ionic strength, but strong charge repulsion at low ionic strength gives rise to an insurmountable barrier that diminishes effective collision. Chemicals and instruments All chemical reagents were obtained from commercial suppliers and used without further purification. Diblock copolymer PSPAA (PS 154 - b -PAA 60 , M n =16,000 for the polystyrene block and M n =4,300 for the poly(acrylic acid) block; M w / M n =1.15) was obtained from Polymer Source; Ligand 1 was purchased from Aldrich; Ligand 2 was purchased from Avanti Polar Lipids; DMF (99.8%) was purchased from Tedia Company. Deionized water (resistance >18 MΩ cm −1 ) was used in all of our reactions. All other chemicals were purchased from Sigma-Aldrich. TEM images were collected from a JEM-1400 Transmission Electron Microscope (JEOL) operated at 120 kV. UV–visible spectra were collected on a Cary 100 UV-Vis spectrophotometer. Preparation of TEM samples (NH 4 ) 6 Mo 7 O 24 was used as a negative stain (3.4 mM) in all TEM images reported in this paper, so that polymer shells appeared white against a dark background. TEM grids were treated by oxygen plasma in a Harrick plasma cleaner/sterilizer for 1 min to improve the surface hydrophilicity. A sample solution was carefully mixed with stain solution on the surface of a plastic Petridish, forming a small bead; a TEM grid was then floated on the top of the bead with the hydrophilic face contacting the solution. The TEM grid was then carefully picked up by a pair of tweezers, wicked with filter paper to remove excess solution and finally dried in air for 20 min. Synthesis of AuNPs Two different size of sodium citrate-stabilized AuNPs (18 nm (ref. 35 ) and 36 nm (ref. 36 )) were prepared based on the literature reports with small modifications (more details available in Supplementary Information ). Synthesis of A-NPs (1-AuNPs) First, 1.5 ml citrate-AuNPs ( d AuNP =18 nm) was concentrated to 100 μl by centrifugation at 13,300 g for 15 min. Then the AuNPs solution was added dropwise to 300 μl of 1 in ethanol (4 mg ml −1 ). The mixture was incubated for 2 h. Then, the A-NPs were purified twice by centrifugation in DMF to remove the excess 1 . These solutions were typically used within 15 min, otherwise partial ligand dissociation can lead to aggregation of the A-NPs. Preparation of B-NPs solution B-NPs solution was prepared by concentrating the citrate-AuNPs solution and re-dispersing the NPs in water to remove the excess Na 3 citrate from the as-synthesized solution. Setup of the nanoreactions The salt concentrations in the B-NPs solution were carefully controlled in the reactions using the synthesis of AB 2 nanoclusters as an example here (details for the syntheses of other AB n nanoclusters can be found in the Supplementary Methods ): citrate-AuNPs (3 ml, d AuNP =18 nm) were concentrated to 20 μl by centrifugation at 13,300 g for 15 min and then diluted by adding 180 μl H 2 O. The residue [Na 3 citrate] was estimated to be 98.9 μM and [B]=24.3 nM (in number of NPs). All other conditions were the same: the purified A-NPs in DMF (100 μl, d AuNP =18 nm, [A]=3.04 nM) were slowly added to an aqueous solution containing large excess of B-NPs (200 μl). During the addition, the Eppendorf tube was vortexed to ensure adequate mixing. The reactions are considered to be completed after the mixing; further incubation of the mixture did not alter the results. Polymer encapsulation of the reaction products A volume of 740 μl DMF was added to the reaction mixture, which contains 100 μl DMF and 200 μl H 2 O, followed by 60 μl PS 154 PAA 60 in DMF (8 mg ml −1 ) (refs [6] , [25] ). Finally, 40 μl of 2 in ethanol (2 mg ml −1 ) was added. The mixture was heated to 100 °C for 2 h and then slowly cooled in the oil bath until it reached room temperature. To isolate the nanoclusters from the excess reactants and empty PSPAA micelles, the product solution was diluted (200 μl diluted by 1,300 μl aq. NaOH (pH=10)), and then centrifuged at 13,300 g (or 5,200 g when 36 nm B-NPs were used) for 20 min to remove the supernatant. The collected purplish-red product at the bottom of centrifuge tubes was diluted by 100 μl aq. NaOH (pH=10), giving a stable solution that contained mainly AB n @PSPAA and B@PSPAA. Purification of AB n @PSPAA nanoclusters ( n =2–4) In a typical separation, the mixture of AB n @PSPAA and B@PSPAA (100 μl) was carefully layered on the top of 1,000 μl saturated CsCl solution in an Eppendorf tube, and the tube was centrifuged at 2,300 g for 25 min (ref. 24 ). The resulting solution showed two distinct bands of red and blue colour, separated by a gap. The lower band was extracted, diluted by aq. NaOH (pH=10) and then centrifuged again to remove the excess CsCl. Purification of AB n @PSPAA nanoclusters ( n =1, 2) The collected AB 2 @PSPAA and B@PSPAA mixture in aq. NaOH (pH=10; 100 μl) was added to 800 μl sodium citrate (1.161 mM), followed by 400 μl AgNO 3 (1 mM). Then, 400 μl ascorbic acid (2 mM) was added and the mixture was incubated for 2 h on a shaker. The mixture solution was purified three times by centrifugation at 1,400 g for 15 min and the supernatant containing the unaffected B@PSPAA were removed. The concentrated brown solution was added to 1,000 μl NH 3 ·H 2 O to etch the Ag blocks and the mixture was incubated in an orbital shaker for 12 h with exposure to air. Finally, the purified AB 2 @PSPAA nanoclusters were collected by centrifugation at 2,200 g for 15 min. The purification of AB@PSPAA ( d A =18 nm, d B =36 nm) was similar as that for AB 2 nanoclusters, except that different centrifugation speeds were used. After Ag growth on the surface of the AB nanoclusters, the resulting solution was purified three times by centrifugation at 200 g for 20 min. The etching step was repeated once. Finally, the purified AB@PSPAA were collected by centrifugation at 2,200 g for 20 min. How to cite this article: Wang, Y. et al . A systems approach towards the stoichiometry-controlled hetero-assembly of nanoparticles. Nat. Commun. 1:87 doi: 10.1038/ncomms1089 (2010).